Infection-induced type I interferons activate CD11b on B-1 cells for subsequent lymph node accumulation Innate-like B-1a lymphocytes rapidly redistribute to regional mediastinal lymph nodes (MedLNs) during influenza infection to generate protective IgM. Here we demonstrate that influenza infection-induced type I interferons directly stimulate body cavity B-1 cells and are a necessary signal required for B-1 cell accumulation in MedLNs. Vascular mimetic flow chamber studies show that type I interferons increase ligand-mediated B-1 cell adhesion under shear stress by inducing high-affinity conformation shifts of surface-expressed integrins. In vivo trafficking experiments identify CD11b as the non-redundant, interferon-activated integrin required for B-1 cell accumulation in MedLNs. Thus, CD11b on B-1 cells senses infection-induced innate signals and facilitates their rapid sequester into secondary lymphoid tissues, thereby regulating the accumulation of polyreactive IgM producers at sites of infection. Innate lymphocytes are increasingly recognized in regulating adaptive immunity and as enforcers of lymph node-protective barrier function. Lymphocytes with innate-like characteristics, including ILC’s (NK cells, LTi among others) [1] but also T cells (γδ and NKT) [2] , [3] and B cells (marginal zone and B-1) [4] , [5] , differ from conventional lymphocytes in both their surface markers and behaviour, and support adaptive immune mechanisms in multiple ways [6] , [7] , [8] , [9] . Cooperation among a spatially clustered network of innate-like cells within the lymph node can regulate macrophage populations, leading to antimicrobial resistance and protection against lymph-borne infection [10] , emphasizing the importance of efficient recruitment and arrangement of innate-like cells within lymph nodes for host defense. Identifying specific mechanisms by which innate-like lymphocytes are activated and positioned is central to understanding their function and eventual clinical manipulation. B-1 cells are innate-like participants in immune responses within secondary lymphoid tissues. They are phenotypically distinguished into two daughter populations: CD5+ B-1a and CD5− B-1b cells [11] . B-1 cells differ in development, tissue location and function from conventional B cells, and have possible functional homologues in humans [5] , [12] . In steady state, splenic and bone marrow B-1 cells are a main source of natural antibody [13] . Natural antibody is polyreactive, mediates tissue integrity and homeostasis by binding self-antigens on apoptotic cells for clearance [14] , and targets a wide variety of pathogens for neutralization including influenza virus, Vaccina virus, Vesticular Stomatitis Virus, Lymphocytic choriomeningitis virus (LCMV), Listeria, Rotavirus and Enterobacter coli and Enterobacter coloace [6] , [15] . In response to pathogenic insult, B-1 cells move from their primary location within the peritoneal and pleural cavities to secondary lymphoid tissues such as the spleen and lymph nodes and begin to secrete IgM. Early studies traced the appearance of peritoneal-origin B-1 cells to the mesenteric lymph nodes or intestinal lamina propria following transfer into lethally irradiated mice [16] , [17] and following their activation by mitogen, antigens or cytokines into the spleen [18] , [19] . Following influenza virus infection, B-1 cells redistribute to regional mediastinal lymph nodes (MedLN) to become a primary source of locally secreted IgM [20] . Thus, the accumulation of B-1 cells in secondary mucosal lymphoid organs and their subsequent differentiation to antibody-secreting cells (ASC) is a common outcome of their activation. However, the precise mechanisms activating B-1 cells to migrate to these sites remain ill defined. CXCL13 is required for B-1 cell migration to and from the peritoneal cavity [21] , [22] , whereas upregulation of CXCR4 and corresponding CXCL12 responsiveness following lipopolysaccharide (LPS) stimulation induced the efflux of B-1 cells from the peritoneal cavity [23] . Others showed a MyD88-dependent decrease in peritoneal B-1 cell frequencies in response to the introduction of intestinal bacteria or LPS into that site and an increase in B-1 cells in the omentum and mesenteric lymphoid tissues. Ha et al. attributed this to decreased surface expression of integrins and CD9 (ref. 24 ). Thus, inflammatory signals seem to drive B-1 cells from body cavities to secondary lymphoid tissues, but which signals may facilitate the subsequent sequestration of B-1 cells into secondary lymphoid tissues remains unknown. Most body cavity B-1 cells express the integrin CD11a and CD11b/CD18 (Mac-1/CR3) [25] . The latter is typically absent on other lymphocytes and on B-1 cells in non-cavity sites but is expressed by monocytic and granulocytic lineage cells and by NK cells. CD11b is expressed in a non-activate conformation and mediates leukocyte adhesion and chemotaxis following cell activation during inflammatory responses [26] . While the selective expression of CD11b suggests its role in regulating B-1 cell migration, CD11b gene-targeted mice have normal numbers of peritoneal cavity B-1 cells. We aimed to determine the mechanisms underlying B-1 cell accumulation in secondary lymphoid tissues by studying their redistribution to regional MedLN following influenza infection, which we had previously demonstrated to occur in an antigen-independent manner and without clonal expansion [20] . Our data demonstrate that direct type I IFNR signalling leads to the preferential accumulation of B-1 cells in MedLN that is facilitated by the activation of CD11b to a high-affinity state, which increased cell adhesion. Activation of CD11b on body cavity B-1 cells by a gradient of innate cytokines, elaborated in response to a local infection, thus facilitates the rapid accumulation of these innate effectors to inflamed lymph nodes, revealing a non-redundant function for CD11b on body cavity B-1 cells and a novel regulatory function for Type I interferon (IFN). B-1a cells accumulate in virus-activated MedLN lymph nodes B-1 cells are the predominant source of IgM in the bronchoalveolar lavage fluid before infection and B-1a cells contribute roughly half of the early-induced IgM in the draining MedLN between days 7 and 10 following influenza virus infection. This B-1a cell contribution occurs in the absence of both appreciable clonal expansion and B-cell receptor-mediated antigen-specific signalling, suggesting innate signals as drivers of the response [20] . To understand the mechanisms by which B-1a cells are drawn to the site of infection, we determined the kinetics with which infection-induced antigen-independent signals activate B-1 cells to accumulate within MedLN. MedLNs are unidentifiably small in wild-type C57BL/6 mice until about 36 h post infection with Influenza A/Mem71. Once clearly visible, MedLNs contain ∼ 1 × 10 6 cells per mouse, increasing to ∼ 1 × 10 7 cells per mouse by day 7 of infection [27] . B-1a cell frequencies, quantified using multicolour flow cytometry ( Supplementary Fig. 1 ), demonstrated that MedLN frequencies exceeded those in peripheral inguinal and axillary lymph nodes (PLN) of the same mice at all time points ( Fig. 1a ). Moreover, by day 7 of infection, B-1 cell-derived IgM-secreting cells, both non-virus-specific IgM secretors and virus-specific IgM secretors, are present at increased numbers in the draining lymph nodes, as demonstrated with neonatal Ig-allotype chimeric mice, in which B-1 and B-2 cells and the IgM they secrete are distinguishable by the Ig-allotype they express [28] ( Fig. 1b ). Together with the nearly 10-fold increases in MedLN cellularity compared with pre-infection levels, this demonstrated an early and selective accumulation of B-1a cells in the MedLN after influenza virus infection as shown previously [20] . 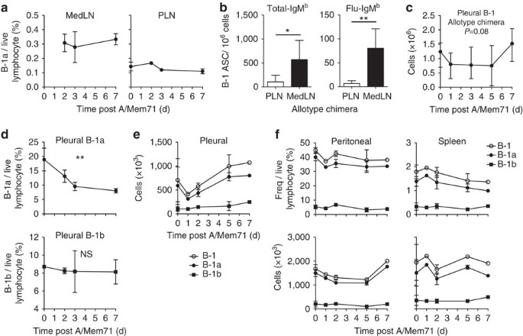Figure 1: Infection-induced accumulation of B-1 cells in MedLN. (a) Flow cytometric analysis of B-1a cell frequency (±s.d.) in lymph nodes of C57BL/6 mice following influenza A/Mem71 infection. PLN, peripheral (inguinal) lymph node. Tissue comparison between MedLN and PLN isP<0.0001 by two-way analysis of variance (ANOVA) for days 2, 3 and 7. SeeSupplementary Fig. 1for gating strategy. (b) ELISpot assay of B-1-derived cells secreting total-IgMband influenza-specific IgMbin MedLN 7 days after infection of Ig-allotype chimeric mice. ASC, antibody-secreting cells. (c) Populations (±s.d.) of B-1 cells in the pleural cavity of Ig-allotype chimeras or pleural (d,e), peritoneal or spleen (f) of C57BL/6 following infection as assessed using flow cytometry. Student’st-test (b) or one- (c,d) or two-way ANOVA (a). n.s., not significant; *P≤0.05, **P≤0.01. Data represent four pooled (a,e,f), two representative (d) or one experiment (b,c). Figure 1: Infection-induced accumulation of B-1 cells in MedLN. ( a ) Flow cytometric analysis of B-1a cell frequency (±s.d.) in lymph nodes of C57BL/6 mice following influenza A/Mem71 infection. PLN, peripheral (inguinal) lymph node. Tissue comparison between MedLN and PLN is P <0.0001 by two-way analysis of variance (ANOVA) for days 2, 3 and 7. See Supplementary Fig. 1 for gating strategy. ( b ) ELISpot assay of B-1-derived cells secreting total-IgM b and influenza-specific IgM b in MedLN 7 days after infection of Ig-allotype chimeric mice. ASC, antibody-secreting cells. ( c ) Populations (±s.d.) of B-1 cells in the pleural cavity of Ig-allotype chimeras or pleural ( d , e ), peritoneal or spleen ( f ) of C57BL/6 following infection as assessed using flow cytometry. Student’s t -test ( b ) or one- ( c , d ) or two-way ANOVA ( a ). n.s., not significant; * P ≤0.05, ** P ≤0.01. Data represent four pooled ( a , e , f ), two representative ( d ) or one experiment ( b , c ). Full size image Infection increases B-1 cell efflux from pleural cavities B-1a cell accumulation in MedLN following influenza virus infection occurs without appreciable B-1a cell proliferation, suggesting rapid B-1 cell redistribution. A tissue-specific decline in total numbers of B-1 cells was observed in the pleural cavity of neonatal Ig-allotype chimeras shortly after infection. Since these cells were identified by Ig-allotype expression, this reduction was not due to changes in surface phenotype ( Fig. 1c ). Reduced B-1a cell frequencies and numbers in the pleural cavity of wild-type mice were observed as early as 2 days following infection ( Fig. 1d,e ) and corresponded chronologically with the accumulation of B-1a cells in the nearby MedLN. Although there is a clear selective reduction in B-1 cell frequencies, the reduction in absolute B-1a cell numbers is more modest, possibly because of changes in distribution of B-1a cells that might include both influx and efflux at the pleural cavity site. The lack of changes in B-1b cell frequencies in the pleural cavity ( Fig. 1d ) was consistent with the previously observed lack of B-1b cell accumulation in the MedLN after influenza infection [20] . No changes were observed in the frequency or number of peritoneal cavity or spleen B-1a cells ( Fig. 1f ). Thus, influenza infection induces a net efflux of B-1a cells from pleural but not peritoneal cavities. Next, we investigated the degree of B-1 cell repositioning between the pleural cavity and draining lymph nodes following influenza infection. Injection of Indium-111-radiolabelled B-1 cells into the pleural cavity of mice that were concurrently virally or mock-infected confirmed a much more drastic reduction in pleural B-1 cells following A/Mem71 infection compared with mock-infected mice, as assessed with full-body autoradiography ( Fig. 2a ). Radioactivity was detected in MedLN but not PLN 3 days after influenza infection but not after mock infection ( Fig. 2a , right panel), indicating a repositioning of pleural cavity B-1 cells to the MedLN. Similar results were obtained when B-1 cells labelled with e670 were injected directly into the pleural cavity on the day of infection and their migration assessed using flow cytometry 3 days after transfer ( Fig. 2b and Supplementary Fig. 2a,b ). At that time, labelled B-1a cells were identified in the MedLN of infected mice at increased frequency compared with uninfected controls ( Fig. 2b ) and in the MedLN compared with the PLN, where recruitment was hardly detectable above the steady state ( Fig. 2b ). However, only a fraction of the accumulating B-1 cells were labelled, indicating the continued recruitment of unlabelled B-1 cells from endogenous pools either within or outside of the pleural cavity. Labelled B-1a cells in the pleural cavity of infected but not of control mice declined within 24 h after cell transfer in most experiments; however, this reduction did not reach statistical significance. The finding that labelled pleural cavity-origin B-1 cells were identified within the MedLN 3 days after infection are analogous to studies demonstrating the rapid migration of peritoneal cavity B-1 cells to the spleen following intraperitoneal (i.p.) injection of LPS or bacteria [5] , [29] . Thus, body cavity B-1 cells are compartmentalized and rapidly respond to regional insults in organs within each body compartment with migration to regional secondary lymphoid tissues. 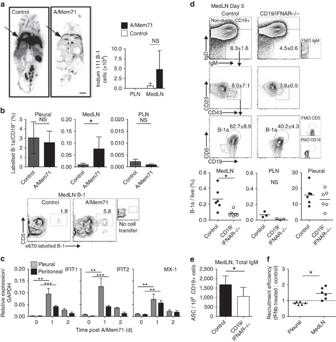Figure 2: B-1 cell redistribution in response to infection-induced signals. (a) Left, full-body autoradiography of mice injected intrapleurally (arrow) with Indium-111-labelled B-1 cells 3 days after A/Mem71 or mock infection. Scale bar, 0.5 cm. Right, gamma scintillation counts of lymph nodes converted to cell numbers using a standard curve developed from Indium-111-labelled B-1 cells (mean (±s.d.). (b) Top, frequency (±s.d.) of e670-labelled pleural cavity and lymph node B-1a cells in C57BL/6 mice 3 days after infection and intrapleural labelled B-1 cell transfer. Bottom, representative contour plots (n=4 mice per group) identify e670+ B-1a cells in MedLN. (c) qRT–PCR analysis of gene expression among purified cavity B-1a cells following infection. The mean (±s.d.) of three samples per time point, each from pooled B-1a cells (n=12 mice). (d) Top, B-1a cell contour plot gating in MedLN from CD19/IFNAR−/− mice and littermate controls 5 days following infection. Bottom, day-5 tissue B-1a cell frequencies using flow cytometry. Each symbol represents one mouse; horizontal line indicates the mean. (e) The mean numbers (±s.d.) IgM-secreting cells (ASC) in MedLN of CD19/IFNAR−/− mice and littermate controls day 5 after A/Mem71 infection. (f) Competition assay comparing tissue recruitment of autoMAC-purified B-1 cells from cavities of C57BL/6 mice labelled with CFSE or e670-tracking dyes, cultured with IFN-β, washed, mixed at even proportions and transferred to the pleural cavity ofn=6 C57BL/6 mice 4 days after infection. Tissue B-1a cells identified using flow cytometry 3 days after transfer (Day 7 post infection). Data presented as recruitment efficiency of labelled B-1a cells compared with controls based on tracking dye ratio normalized to input ratio. MedLN recruitment efficiency was significant compared with value of 1.0 by one samplet-test (P=0.02). A similar experiment conducted using Ig-allotype to distinguish between groups of transferred cells showed comparable results (Supplementary Fig. 2c). Student’st-test: n.s., not significant; *P≤0.05, **P≤0.01, ***P≤0.001. Data represent one experiment (a,f), five experiments (b), two experiments (Ifit1andIfit2) one experiment (Mx-1;c) or two pooled experiments (d,e). Figure 2: B-1 cell redistribution in response to infection-induced signals. ( a ) Left, full-body autoradiography of mice injected intrapleurally (arrow) with Indium-111-labelled B-1 cells 3 days after A/Mem71 or mock infection. Scale bar, 0.5 cm. Right, gamma scintillation counts of lymph nodes converted to cell numbers using a standard curve developed from Indium-111-labelled B-1 cells (mean (±s.d.). ( b ) Top, frequency (±s.d.) of e670-labelled pleural cavity and lymph node B-1a cells in C57BL/6 mice 3 days after infection and intrapleural labelled B-1 cell transfer. Bottom, representative contour plots ( n =4 mice per group) identify e670+ B-1a cells in MedLN. ( c ) qRT–PCR analysis of gene expression among purified cavity B-1a cells following infection. The mean (±s.d.) of three samples per time point, each from pooled B-1a cells ( n =12 mice). ( d ) Top, B-1a cell contour plot gating in MedLN from CD19/IFNAR−/− mice and littermate controls 5 days following infection. Bottom, day-5 tissue B-1a cell frequencies using flow cytometry. Each symbol represents one mouse; horizontal line indicates the mean. ( e ) The mean numbers (±s.d.) IgM-secreting cells (ASC) in MedLN of CD19/IFNAR−/− mice and littermate controls day 5 after A/Mem71 infection. ( f ) Competition assay comparing tissue recruitment of autoMAC-purified B-1 cells from cavities of C57BL/6 mice labelled with CFSE or e670-tracking dyes, cultured with IFN-β, washed, mixed at even proportions and transferred to the pleural cavity of n =6 C57BL/6 mice 4 days after infection. Tissue B-1a cells identified using flow cytometry 3 days after transfer (Day 7 post infection). Data presented as recruitment efficiency of labelled B-1a cells compared with controls based on tracking dye ratio normalized to input ratio. MedLN recruitment efficiency was significant compared with value of 1.0 by one sample t -test ( P =0.02). A similar experiment conducted using Ig-allotype to distinguish between groups of transferred cells showed comparable results ( Supplementary Fig. 2c ). Student’s t -test: n.s., not significant; * P ≤0.05, ** P ≤0.01, *** P ≤0.001. Data represent one experiment ( a , f ), five experiments ( b ), two experiments ( Ifit1 and Ifit2 ) one experiment ( Mx-1 ; c ) or two pooled experiments ( d , e ). Full size image B-1a cell MedLN accumulation requires Type I IFN signalling Type I IFN is a common downstream effector of TLR-3, 7, RIG-I and Mda-5 signals, all involved in innate viral recognition [30] , [31] , and rapidly stimulates follicular B cells in MedLN after influenza infection [32] . Similarly, 1 day after infection, pleural and peritoneal cavity B-1 cells showed increased expression of numerous Type I IFN-regulated genes, including Ifit1 , Ifit2 and Mx1 among others ( Fig. 2c ). Expression changes were stronger in pleural compared with peritoneal cavity B-1 cells, consistent with initial virus-induced local type I IFN secretion, followed by a systemic spread [32] , [33] . Notably, B-1a cell frequencies in MedLN of B-cell-specific type I IFNR-deficient mice (CD19/IFNAR−/−) [34] were significantly smaller compared with control animals on day 5 following influenza virus infection, and in fact comparable to those in the non-draining PLN ( Fig. 2d ). Consistent with this, numbers of IgM antibody-forming cells (ASC) in CD19/IFNAR−/− MedLN on day 7 of infection were diminished compared with controls, as assessed using IgM-ELISPOT assays ( Fig. 2e ). In contrast, frequencies of pleural cavity B-1a cells were comparable between control animals and CD19/IFNAR−/− on day 5 after infection ( Fig. 2d ). Thus, type I IFN provides a necessary direct signal for enhanced B-1a cell accumulation in MedLN, but not their enhanced egress from the pleural cavity after influenza infection. We next sought to investigate whether the relationship between type I IFN signalling and accumulation of B-1a cells required other cell types or was a direct effect on B-1 cells. For that, we compared MedLN recruitment of B-1a cells cultured with type I IFN or medium alone before intrapleural transfer into mice infected for 4 days with Influenza virus. Day 4 of infection was chosen as MedLNs are close to maximally expanded at that time ( Fig. 1a ), yet type I IFN signalling induced by the infection is close to pre-infection levels. Three days after adoptive transfer (day 7 post infection), labelled B-1a cells were identified in various tissues and the ratio of migrating B-1a cells from each culture group was compared with their input ratio using flow cytometry ( Supplementary Fig. 2c ). The data clearly showed that B-1 cells pre-treated with IFN-β accumulated more efficiently in the MedLN than non-stimulated B-1 cells, while their frequencies in the pleural cavity and blood remained comparable ( Fig. 2f ). Thus, Type I IFNR direct signalling regulates B-1 cell redistribution from body cavities to secondary lymphoid tissues. Infection-induced type I IFN increases B-1 cell adhesion To determine the mechanisms of IFN-facilitated accumulation of B-1a cells within the draining MedLN in response to viral infection, we optimized a microfluidic vascular mimetic flow chamber system for use with B-1 cells [35] ( Fig. 3a ). Numerous integrin and chemokine combinations were tested for induction of body cavity B-1 cell adhesion and arrest under shear stress. ICAM-1 and CXCL13 were identified to facilitate low-level arrest before B-1 cell stimulation and strong arrest following B-1 cell stimulation through G-protein-coupled receptor agonist N-formyl-methionyl-leucyl-phenylalanine (fMLP; Fig. 3b ). Importantly, in vivo influenza infection-induced signals dramatically increased the adhesion behaviour of pleural but not peritoneal cavity B-1 cells isolated from those sites at 24 and 48 h after infection ( Fig. 3c ). 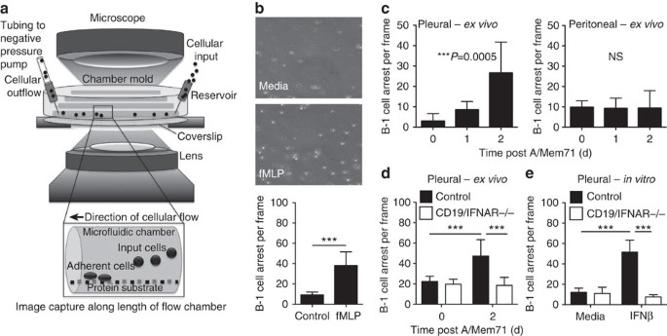Figure 3: Infection-induced type I IFN signalling increases B-1 cell integrin-mediated adhesion. (a) Schematic of a vascular mimetic microfluidic chamber used to observe adhesion of B-1 cells on cover slips coated with ICAM-1 and CXCL13 under shear flow. (b) 20 × brightfield images of autoMACS-purified B-1 cells in the medium without (top) or with (bottom) 1 μM fMLP. Bar chart shows the mean B-1 cells arresting (±s.d.). (c) Adhesion assay showing the mean numbers (±s.d.) of pleural and peritoneal cavity B-1 cell arrests by B-1 cells isolated from mice at indicated times of infection with A/Mem71. (d) As inc, with B-1 cells isolated from CD19/IFNAR−/− mice and littermate controls. (e) As ind, with cells stimulatedin vitrowith 200 U IFN-β for 16 h. Student’st-test: n. s., not significant; ***P≤0.001. Data representative of three (a) or two (b–d) separate experiments. In each experiment, purified B-1 cell samples for adhesion studies were pooled fromn=12 mice per group. Figure 3: Infection-induced type I IFN signalling increases B-1 cell integrin-mediated adhesion. ( a ) Schematic of a vascular mimetic microfluidic chamber used to observe adhesion of B-1 cells on cover slips coated with ICAM-1 and CXCL13 under shear flow. ( b ) 20 × brightfield images of autoMACS-purified B-1 cells in the medium without (top) or with (bottom) 1 μM fMLP. Bar chart shows the mean B-1 cells arresting (±s.d.). ( c ) Adhesion assay showing the mean numbers (±s.d.) of pleural and peritoneal cavity B-1 cell arrests by B-1 cells isolated from mice at indicated times of infection with A/Mem71. ( d ) As in c , with B-1 cells isolated from CD19/IFNAR−/− mice and littermate controls. ( e ) As in d , with cells stimulated in vitro with 200 U IFN-β for 16 h. Student’s t -test: n. s., not significant; *** P ≤0.001. Data representative of three ( a ) or two ( b – d ) separate experiments. In each experiment, purified B-1 cell samples for adhesion studies were pooled from n =12 mice per group. Full size image Consistent with the in vivo findings ( Fig. 2f ), direct type I IFNR signalling was necessary for the increased B-1 cell adhesion ex vivo , as B-1 cells from 2-day influenza-infected CD19/IFNAR−/− mice lacked increased adhesion properties ( Fig. 3d ). Furthermore, in vitro treatment with IFN-β of pleural cavity B-1 cells from non-infected controls, but not CD19/IFNAR−/− mice, stimulated increased adhesion at levels equivalent to those seen with B-1 cells ex vivo after infection, showing that direct type I IFN-signalling is sufficient to increase B-1 cell adhesion to ICAM-1/CXCL13 ( Fig. 3e ). Together, these results indicated that pleural B-1 cells receive a sufficiently strong infection-induced IFN signal in vivo to alter their adhesion properties to a chemokine and/or integrin substrate, which may account for their increased ability to enter into activated lymphoid tissues. Type I IFN B-1 cell activation is chemokine-independent We investigated the effects of type I IFN on B-1 cell chemokine receptor surface expression and receptor sensitivity. CXCL13 guides B-1 cell movement into the peritoneal cavity [21] , [24] and its receptor, CXCR5, is highly expressed on B-1 cells [21] . B-1a cells in various tissues expressed CXCR5 before influenza infection, and their expression levels roughly doubled in MedLN, PLN and in the pleural but not the peritoneal cavities 2 days following influenza infection ( Supplementary Fig. 3a ). B-1 cell migration towards CXCL13, however, was not altered by type I IFN pre-treatment, indicating that the modest increases in CXCR5 expression did not increase their chemotactic responses ( Supplementary Fig. 3b ). Furthermore, addition of a CXCL13-blocking antibody to the vascular mimetic flow chamber reservoir before introducing wild-type or CD19/IFNAR−/− B-1 cells stimulated with type I IFN did not affect their arrest ( Supplementary Fig. 3c ), while it completely blocked chemotaxis ( Supplementary Fig. 3b ). Thus, type I IFN induced B-1 cells are activated and arrest independently of CXCL13-mediated chemotactic signals. CD11b-dependent migration of type I IFN-activated B-1 cells All B-1 cells express the integrin CD11a, but body cavity B-1 cells are unique in that they, but not their counterparts in lymphoid tissues, also express CD11b/CD18 (ref. 25 ). Integrin-mediated adhesion of lymphocytes regulates their tissue redistribution in the steady state, and ICAM-1 serves as a substrate for CD11a (LFA-1) and CD11b (Mac-1). To determine the role of integrins in type I IFN-induced recruitment of B-1 cells to tissue sites following infection, we expanded our earlier competition study ( Fig. 2f ) to evaluate migration of IFN-β-activated B-1 cells exposed to Lovastatin, an inhibitor of integrin-dependent leukocyte adhesion [37] . Purified B-1 cells from IgM a and IgM b allotype mice were treated with IFN-β overnight. IgM a -allotype B-1 cells were subsequently treated in addition with Lovastatin for 10 min, washed and then combined in equal proportion with IgM b B-1 cells. Cells were transferred into the pleural cavity of B-cell-deficient μMT mice that were infected 4 days before A/Mem71, and their accumulation into the MedLN assessed 72 h later (day 7 of infection) using flow cytometry. The results revealed that cells treated with IFN-β plus Lovastatin were recruited significantly less frequently to the MedLN compared with cells treated only with IFN-β, while their frequencies in the pleural cavity were if anything increased compared with that of the controls ( Fig. 4a ). The data suggested that integrin activation by type I IFN signalling contributes to the B-1 cell recruitment processes from the pleural cavity into lymphoid tissues following influenza infection. 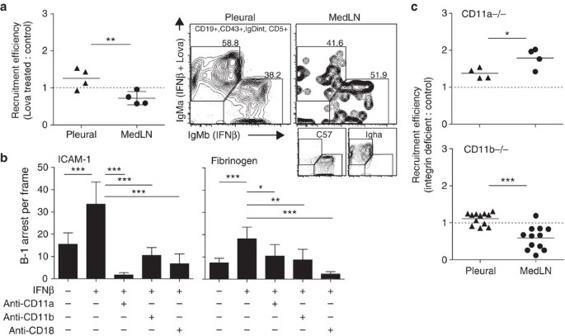Figure 4: Type I IFN activation of CD11b alters B-1 cell adhesion. (a) Competition assay comparing tissue recruitment of autoMAC-purified B-1 cells from body cavities of allotype disparate Igha or C57BL/6 mice cultured with 200 U IFN-β 16 h, ±100 μM Lovastatin 10 min to a-allotype cells, mixed equally and transferred into pleural cavities of μMT mice 4 days after A/Mem71 infection. Tissue B-1a cells were identified by allotype-specific flow cytometry staining 3 days after transfer (Day 7 post infection). Data presented as recruitment efficiency of B-1a cells compared with control cells based on a-/b-allotype ratio normalized to input ratio. Right panel, representative flow cytometry plots showing frequency of allotype B-1 cells from competing groups in the pleural cavity and MedLN at necropsy. MedLN recruitment efficiency was significant compared with the value of 1.0 by one samplet-test (P=0.05). (b) Adhesion assay showing numbers (±s.d.) of the pleural cavity B-1 cell arrest following 16-h stimulation with 200 U IFN-β, measured on ICAM-1 (left) and fibrinogen (right) substrate with or without blocking antibodies against CD11a, CD11b and CD18. (c) Competition assay comparing immigration of separate CFSE or e670-tracking dye-labelled C57BL/6 control and (left) CD11a-deficient or (right) CD11b-deficient cavity cells mixed in even proportions and transferred into the pleural cavity of C57BL/6 mice at the time of infection with A/Mem71. Labelled B-1a cells were identified using flow cytometry staining in MedLN and blood 3 days later. Data are presented as recruitment efficiency of integrin-deficient B-1a cells compared with migration by control cells based on tracking dye ratio normalized to input ratio (Supplementary Fig. 2e). MedLN recruitment efficiency was significant compared with the value of 1.0 by one samplet-test (P=0.009 (CD11a) andP=0.0009 (CD11b)). Data represent one experiment,n=4 mice per group (a,c(CD11a)), two separate experiments for each substrate using pooled pleural cavity B-1 cells isolated fromn>12 mice per group (b) and two pooled experiments,n=4 or 6 mice per group (c(CD11b)). Student’st-test: *P≤0.05, **P≤0.01, ***P≤0.001. Figure 4: Type I IFN activation of CD11b alters B-1 cell adhesion. ( a ) Competition assay comparing tissue recruitment of autoMAC-purified B-1 cells from body cavities of allotype disparate Igha or C57BL/6 mice cultured with 200 U IFN-β 16 h, ±100 μM Lovastatin 10 min to a-allotype cells, mixed equally and transferred into pleural cavities of μMT mice 4 days after A/Mem71 infection. Tissue B-1a cells were identified by allotype-specific flow cytometry staining 3 days after transfer (Day 7 post infection). Data presented as recruitment efficiency of B-1a cells compared with control cells based on a-/b-allotype ratio normalized to input ratio. Right panel, representative flow cytometry plots showing frequency of allotype B-1 cells from competing groups in the pleural cavity and MedLN at necropsy. MedLN recruitment efficiency was significant compared with the value of 1.0 by one sample t -test ( P =0.05). ( b ) Adhesion assay showing numbers (±s.d.) of the pleural cavity B-1 cell arrest following 16-h stimulation with 200 U IFN-β, measured on ICAM-1 (left) and fibrinogen (right) substrate with or without blocking antibodies against CD11a, CD11b and CD18. ( c ) Competition assay comparing immigration of separate CFSE or e670-tracking dye-labelled C57BL/6 control and (left) CD11a-deficient or (right) CD11b-deficient cavity cells mixed in even proportions and transferred into the pleural cavity of C57BL/6 mice at the time of infection with A/Mem71. Labelled B-1a cells were identified using flow cytometry staining in MedLN and blood 3 days later. Data are presented as recruitment efficiency of integrin-deficient B-1a cells compared with migration by control cells based on tracking dye ratio normalized to input ratio ( Supplementary Fig. 2e ). MedLN recruitment efficiency was significant compared with the value of 1.0 by one sample t -test ( P =0.009 (CD11a) and P =0.0009 (CD11b)). Data represent one experiment, n =4 mice per group ( a , c (CD11a)), two separate experiments for each substrate using pooled pleural cavity B-1 cells isolated from n >12 mice per group ( b ) and two pooled experiments, n =4 or 6 mice per group ( c (CD11b)). Student’s t -test: * P ≤0.05, ** P ≤0.01, *** P ≤0.001. Full size image To determine the respective roles of CD11a and CD11b in type I IFN-induced enhanced adhesion of body cavity B-1 cells, we first inhibited integrin-mediated adhesion of B-1 cells in the vascular mimetic chamber, using blocking antibodies against CD11a, CD11b and their shared common beta-2 integrin chain CD18. B-1 cells stimulated with type I IFN increased their ability to arrest on ICAM-1, a ligand for both CD11a and CD11b, but also on fibrinogen, a ligand for CD11b (ref. 26 ). Treatment with various integrin subunit-blocking antibodies abrogated this arrest ( Fig. 4b ). Thus, consistent with the in vivo data ( Fig. 4a ), type I IFN activation of B-1 cell adhesion in vitro was mediated by increased integrin-binding capacity. To further determine whether B-1 cells require integrins to accumulate in MedLN in response to influenza infection, we studied integrin-deficient B-1 cells in vivo . Flow cytometric analysis demonstrated the presence of roughly similar numbers of B-1 cells in the body cavities of CD11a and CD11b gene-targeted mice ( Supplementary Fig. 2d ). Thus neither CD11a nor CD11b are necessary for B-1 cell accumulation in the body cavities. We then used a competition model in which total cavity lavage cells from either CD11a or CD11b-deficient strains were labelled with tracking dyes and injected together with equal numbers of cells from wild-type controls into the pleural cavity of mice ( Supplementary Fig. 2e ), to study the effects of integrin-mediated B-1 cell accumulation in various tissues three days after influenza infection. The results clearly demonstrate that B-1 cells from CD11b−/− animals were at a competitive disadvantage compared to B-1 cells from wild-type mice in attaining MedLN positioning (Fig. 4c ). This difference in the effects of CD11b on the distribution to distinct tissues highlight the particular role for CD11b in facilitating efficient entry of B-1 cells into the lymph nodes, while their exit from the pleural cavity was independent of both type I IFNR-signalling and CD11b function. Somewhat unexpectedly, B-1 cells from CD11a−/− mice appeared to be at a competitive advantage, redistributing to the MedLN at nearly twice the frequency compared to control B-1a cells ( Fig. 4c ). It is possible that in the absence of CD11a, binding via CD11b might be further enhanced, although this will require further study. Taken together we conclude that B-1 cells gain rapid and efficient entry into regional lymph nodes after influenza infection via a mechanism requiring CD11b-integrin-mediated adhesion. CD11b promotes cavity B-1a cell migration to activated MedLN Next, we investigated the mechanisms by which IFNR signals affect CD11b-mediated B-1 cell accumulation after influenza infection. First, we studied expression of CD11a and CD11b on B-1a cells using flow cytometry. As expected, CD11a was highly expressed by lymph node B-1a cells both before and after infection ( Fig. 5a ). Surface expression of CD11a by B-1a cells remained largely unaffected in the MedLN, PLN, pleural and peritoneal cavities at early time points following infection ( Fig. 5a,b ). 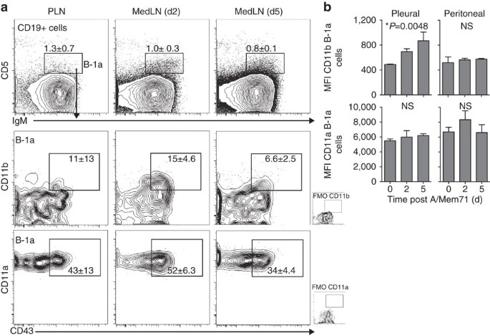Figure 5: CD11b expression by recent B-1 cell lymph node immigrants. (a) Shown are contour plots with outliers of CD11b and CD11a expression after gating for live, non-dump, CD19+ cells (top) and gating for expression of IgM and CD5 to identify B-1a cells (lower panels) among MedLN cells from days 2 and 5 after infection with A/Mem71. Numbers indicate the mean frequencies (±s.d.). FMO, fluorescent minus one control. (b) The mean fluorescence intensity (MFI, ±s.d.) of CD11a and CD11b expression by pleural and peritoneal B-1 cells at indicated times after infection. Student’st-test: n.s., not significant; *P≤0.05. Data are representative of three experiments that gave similar results,n=3 mice per group (a,b). Figure 5: CD11b expression by recent B-1 cell lymph node immigrants. ( a ) Shown are contour plots with outliers of CD11b and CD11a expression after gating for live, non-dump, CD19+ cells (top) and gating for expression of IgM and CD5 to identify B-1a cells (lower panels) among MedLN cells from days 2 and 5 after infection with A/Mem71. Numbers indicate the mean frequencies (±s.d.). FMO, fluorescent minus one control. ( b ) The mean fluorescence intensity (MFI, ±s.d.) of CD11a and CD11b expression by pleural and peritoneal B-1 cells at indicated times after infection. Student’s t -test: n.s., not significant; * P ≤0.05. Data are representative of three experiments that gave similar results, n =3 mice per group ( a , b ). Full size image Lymph node B-1a cells largely lacked expression of CD11b. However, we noted a distinct population of CD11b-expressing B-1 cells in the MedLN on day 2 but not day 5 after infection with influenza virus ( Fig. 5a ), suggesting that B-1a cells downregulate CD11b expression after their entry into the lymph node. This is consistent with studies that demonstrated the early and transient presence of CD11b+ B-1 cells in the spleen of mice injected i.p. with Francisella [36] or LPS [19] . Thus, the unique surface expression of CD11b on body cavity B-1 cells coincides with and facilitates their rapid entry into secondary lymphoid tissues, after which expression is downregulated. After influenza infection, expression of CD11b increased in pleural but not peritoneal cavity B-1 cells ( Fig. 5b ). However, these increases appeared modest. In addition, CD11b expression was comparable in wild-type and CD19/IFNAR−/− mice in multiple tissues ( Fig. 6a ), indicating that, while influenza-induced signals increased CD11b expression by pleural cavity B-1 cells ( Fig. 5b ), they were unlikely solely responsible for the strong increases in B-1 cell adhesion in vitro ( Fig. 3d ). Integrins can alter their tertiary structure to a high-affinity conformation state that stabilizes binding to their ligands. To clarify the relationship between type I IFN and activation of integrins, we treated pleural B-1 cells (isolated from infected animals or pre-treated with IFN-β) with either fMLP to activate the conversion of integrins to their high-affinity conformation, or lovastatin, an inhibitor that stabilizes integrins in a low-affinity state [37] . Body cavity B-1 cells isolated from wild-type mice and subsequently treated with fMLP responded with activation-mediated increased arrest on ICAM-1, confirming that integrin activation also stabilizes B-1 cell arrest ( Fig. 6b,c ). Activation of type I IFNR-deficient pleural cavity B-1 cells with fMLP also induced B-1 cell arrest. However, these cells neither increased adhesion in response to pre-treatment with IFN-β in vitro or following influenza infection in vivo ( Fig. 6b,c ). This demonstrated that IFNAR−/− pleural cavity B-1 cells can be activated via non-IFNR signals to increase integrin-mediated adhesion, but that during influenza infection no other signals are present, at least at the early time points tested ( Fig. 6b,c ). 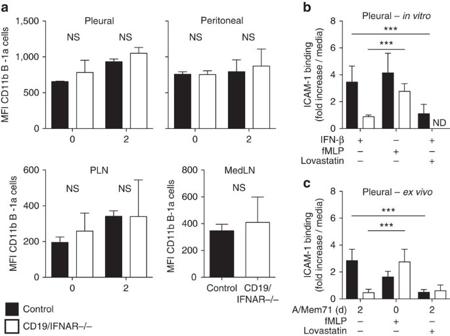Figure 6: Type I IFN alters affinity conformation of CD11b. (a) Shown are the MFIs (±s.d.) of CD11b expression on B-1a cells in pleural (top left) and peritoneal cavity B-1 cells (top right), PLN and MedLN (bottom left and right, respectively) from CD19/IFNAR−/− (open bars) mice and littermate controls (closed bars) at indicated times after infection with A/Mem71. (b) Adhesion assay showing fold inductions of B-1 cell adhesion over media controls in vascular mimetic chambers under shear-flow when stimulatedin vitrofor 16 h with IFN-β, or immediately before fMLP in the presence or absence of lovastatin, an inhibitor of integrin activation. Cells were from wild type (filled bars) or CD19/IFNAR−/− mice (open bars). (c) As inb, pleural cavity B-1 cells were isolated from non-infected or day-2-A/Mem/71-infected mice before exposure to lovastatin. Student’st-test: n.d., not done. n.s., not significant; ***P≤0.001. Data from one experiment (a–c) withn=3 (a) orn=12 pooled (b,c) mice per group. Figure 6: Type I IFN alters affinity conformation of CD11b. ( a ) Shown are the MFIs (±s.d.) of CD11b expression on B-1a cells in pleural (top left) and peritoneal cavity B-1 cells (top right), PLN and MedLN (bottom left and right, respectively) from CD19/IFNAR−/− (open bars) mice and littermate controls (closed bars) at indicated times after infection with A/Mem71. ( b ) Adhesion assay showing fold inductions of B-1 cell adhesion over media controls in vascular mimetic chambers under shear-flow when stimulated in vitro for 16 h with IFN-β, or immediately before fMLP in the presence or absence of lovastatin, an inhibitor of integrin activation. Cells were from wild type (filled bars) or CD19/IFNAR−/− mice (open bars). ( c ) As in b , pleural cavity B-1 cells were isolated from non-infected or day-2-A/Mem/71-infected mice before exposure to lovastatin. Student’s t -test: n.d., not done. n.s., not significant; *** P ≤0.001. Data from one experiment ( a – c ) with n =3 ( a ) or n =12 pooled ( b , c ) mice per group. Full size image Importantly, the addition of the inhibitory agent lovastatin completely reverted the increased IFN-mediated arrest of pleural cavity B-1 cells either following their in vitro stimulation with IFN-β ( Fig. 6b ), or ex vivo following influenza infection ( Fig. 6c ). These data demonstrate a non-redundant function for type I IFN in triggering a high-affinity conformation state for integrins on pleural cavity B-1 cells following influenza virus infection, of which we show CD11b to be required for efficient recruitment of B-1a cells into the MedLN after influenza infection and their subsequent contributions to the production of local IgM. Lymph nodes are important domains of adaptive immune response induction that rapidly increase in cellularity following a local insult/infection. T- and B-cell accumulation is driven by increased retention and antigen-driven clonal expansion. In addition, various innate-like lymphocytes accumulate in inflamed LN without extensive proliferation, where they modulate the quality of adaptive immune responses and contribute to the immunological barrier [10] . They may also play pathogenic roles during autoimmune disease induction [38] . This study identifies a novel axis of type I IFN-mediated integrin activation for rapid accumulation of one such innate lymphocyte subset, B-1 cells, in the respiratory tract draining lymph nodes following influenza infection. Type I IFN was shown to act on reservoirs of body cavity B-1 cells to increase integrin-mediated adhesion in vitro and ex vivo . The activation of the integrin CD11b was uniquely required for the accumulation of B-1 cells in the lymph node. As B-1 cells may also provide functions other than IgM secretion, including the secretion of cytokines such as IL-10 (ref. 39 ) or granulocyte–macrophage colony-stimulating factor [40] , [41] , the identification of mechanisms that regulate B-1a cell accumulation may foster discovery of additional B-1 cell roles in immune response regulation. Our studies demonstrate for the first time that integrin activation can be induced by type I IFN. During most viral infections, influenza infection rapidly induces type I IFN by infected epithelial cells and likely stromal cells in regional lymph nodes [42] , [43] , where it directly activates B cells [42] . Type I IFN enhances the magnitude and quality of adaptive B-cell responses to influenza and other viral infections [32] , [42] , [44] . Specifically, Type I IFN inhibits recirculation of lymphocytes from lymph nodes to blood by inducing expression of CD69, which negatively regulates S1P-1 signalling, retaining B and T cells within lymph nodes during immune responses and thereby regulating lymph node size and cell migration [45] , [46] . Thus, it was not surprising to find type I IFN-mediated activation of local B-1 cell populations following influenza infection. However, the mechanisms by which type I IFN acts to cause B-1 cell accumulation are distinct from those described for T and conventional B cells, as it involved activation of the integrin CD11b into an activated, high-affinity state, enhancing the binding to ICAM-1 and IFN-mediated induction of a CD11b high-affinity state was crucial for increased adhesion of B-1 cells to ligands in vitro and their accumulation in MedLN in vivo , while strong expression of CD11a did not significantly affect B-1a cell accumulation. Body cavity B-1 cells, but not counterparts in lymph nodes, bone marrow or spleen express CD11b. Our data point to the selective expression of CD11b on body cavity B-1 cells: readying these cells for rapid redistribution into secondary lymphoid tissues when activated by innate signals. Others have shown that subsets of body cavity B-1 cells lack expression of CD11b [47] , and that CD11b-negative B-1 cells give rise to CD11b-expressing cells after body cavity arrival [48] . Our studies now assign a function to B-1 cell acquisition of CD11b in the body cavity consistent with multiple studies demonstrating migration of peritoneal cavity B-1 cells from body cavities to spleen and lymph nodes after activation with LPS, whole bacteria or various cytokines [5] . Our data further underscore the notion that body cavity B-1 cells represent reservoirs of innate lymphocytes that quickly reposition in response to insult, explain a longstanding puzzle in B-1 cell biology about the significance of CD11b expression and raise interesting questions regarding ‘reservoirs’ of other innate-like lymphocytes, many of which also express CD11b. Although we identified the pleural cavity as a source of MedLN B-1a cells following respiratory tract infection, this does not preclude contributions from other tissues. In that case, pleural-emigrating B-1a cells might only represent a fraction of MedLN B-1a cell populations. On the basis of the emerging data, we favour a model in which B-1 cells slowly but continuously circulate to and from body cavities to peripheral sites even in the absence of inflammation, potentially via the blood, which contains significant numbers of B-1 cells. Our data clearly demonstrate preferential circulation to the MedLN by type I IFN-activated B-1 cells as one mechanism by which the inflammatory response to infection shapes draining lymph node B-1a cell populations. Still, the tissue-specific kinetics of this continuous influx and efflux of travelling B-1 cells in the steady state and in response to inflammatory stimuli require further exploration. Furthermore, the mechanisms that induce CD11b shedding after body cavity exit and its re-expression by B-1 cells following CXCL13-dependent repositioning into body cavities [21] remain to be identified. As integrins are central to the migration of all leukocytes and type I IFN is produced in response to all viruses (and most intracellular bacteria), our findings may contribute to interpretation of immune response alterations in other diseases. For example, recent studies report effects of type I IFN ‘signature’ responses during chronic lymphocytic choriomeningitis virus (LCMV) infection [49] , [50] and in autoimmune diseases such as systemic lupus erythematosus (SLE) [51] . Our results provide new insights into the functions of this cytokine family and its regulation of leukocyte migration, particularly the migration of innate-like lymphocytes, whose contributions to disease pathogenesis are only beginning to be addressed. Mice Groups of 6- to 12-week-old female C57BL/6, MyD88−/−, type I IFNR−/−, CD11a−/−, CD11b−/−, μMT and B6.Cg Igh-a mice (all from Jackson Laboratories, C57BL/6 background), BALB/c mice (Harlan Laboratories) and B-cell-specific type I IFNAR KO (CD19/IFNAR−/−; generated as previously described [34] , C57BL/6 background) mice were purchased or bred and maintained in microisolator cages under conventional housing conditions at UC Davis. Except allotype chimeras, all mice were used between 8 and 12 weeks of age, according to the protocols approved by the UC Davis Animal Use and Care Committee. Neonatal chimeras in which B-1 and B-2 cells are distinguished by Ig-allotype were created according to the published protocols [52] . Specifically, B6.Cg Igh-a pups were treated with anti-IgM-a-allotype monoclonal antibodies (DS1.1) i.p. (0.1 mg in 100 μl PBS 24 h after birth and then 0.2 mg in 100 μl PBS twice weekly for 6 weeks) to deplete all host B cells. Pups were reconstituted by i.p. injection of 100 μl PBS containing 5 × 10 6 pleural and peritoneal lavage cells from C57BL/6 (Igh b ) mice as a source of B-1 cells 48 h after birth. Six weeks following cessation of treatment mice are fully reconstituted: bone marrow-derived B-cell development replenishes peripheral B-2 cells (a-allotype), but not B-1 cells. Thus, Igh-b expression identifies B-1 cells, whereas other B-cell subsets express Igh-a. For validation of approach see ref. 28 . Influenza virus and intranasal infection Mice were anaesthetized with isoflurane and infected intranasally with a sublethal dose (12,000 plaque-forming unit per mouse) of influenza A/Mem71 (Mem71)-containing allantoic fluid in 40-μl sterile PBS and killed 2–10 days later. Mem71 is a reassortant influenza virus strain carrying the haemagglutinin of A/Memphis/1/71(H3) and the neuraminidase of A/Bellamy/41(N1). Virus preparation was conducted as previously described [53] . Flow cytometry For flow cytometric analysis, B-1a cells were stained as previously described [53] with Fc block (2.4.G2, 5 μg ml −l ) followed by the following antibody conjugate panels at concentrations predetermined to be optimal for each batch by titration. Antibodies were in-house generated from indicated clone unless otherwise noted: CD5-Biotin (53–7.8), Streptavidin (SA)-QDOT605A (Thermo Fischer Q10101MP), CD23-FITC (B3B4.2), CD43-PE (S7), CD90.2-Cy5PE (Thy1.2, 30H12) or CD4-Cy5PE (GK1.5), CD8a-Cy5PE (53–6.7), CD3-Cy5PE (145-2C11) and Gr-1-Cy5PE (RB6-8c5), F4/80-Cy5PE (F4/80), CD49b (PanNK)-Cy5PE (DX-5, BioLegend 108901 or PK136), IgD-Cy7PE (11-26c), CD19-APC (1D3) and IgM-Alexa700 (331) ( Supplementary Fig. 1 ). Chemokine panel: CXCR5-biotin (2G8, eBiosciences, 13–7185), SA-QDOT (Thermo Fisher, Q10101MP), CD90.2-PacBlue (Thy1.2, 30H12), Gr-1-PacBlue (RB6-8c5), F4/80-PacBlue (F4/80), CD49b-PacBlue (DX-5, BioLegend 108901), CD23-FITC (B3B4.2, BD), CD5-PE (53-7.8), CD19-Cy5PE (1D3), CD43-Cy5.5PE (S7), IgD-Cy7PE (11-26c), CXCR4-APC (2B11, eBiosciences 17-9991) and IgM-Alexa700 (331). Integrin panel: CD5-Biotin (53–7.8), Streptavidin (SA)-QDOT605A (Thermo Fischer Q10101MP), CD90.2-PacBlue (Thy1.2, 30H12), Gr-1-PacBlue (RB6–8c5), F4/80-PacBlue (F4/80), CD49b-PacBlue (DX-5, BioLegend 108901), CD23-FITC (B3B4.2), CD43-PE (S7), CD11b-Cy5PE (Mac1.13), CD11a-Cy7PE (2D7), CD19-APC (1D3) and IgM-Alexa700 (331). Chimera panel: CD5-Biotin (53–7.8), SA-QDOT605A (Thermo Fischer Q10101MP), CD4-PacBlue (GK1.5), CD8a-PacBlue (53–6.7), CD3-PacBlue (145-2C11), Gr-1-PacBlue (RB6-8c5) and F4/80-PacBlue (F4/80), CD49b-Pacblue (DX-5, BioLegend 108901), CD23-FITC (B3B4.2), CD19-Cy5PE (1D3), CD43-Cy7APC (S7), IgD-Cy7PE (11-26c), IgM a -APC (DS1.1) and IgM b -PE (AF6-78). In all panels, Live Dead Violet (Thermo Fischer L34955) was used to discriminate non-viable cells. Data were acquired using a FACS Aria (BD) equipped with lasers and optics for 13-colour data acquisition. Data were analyzed using the FlowJo software (gift of A. Treestar, Tree Star Inc.). ELISpot Total and virus-specific IgM-secreting antibody-forming cells (ASC) were enumerated using ELISpot as described [53] . Briefly, 96-well plates (Multi-screen HA Filtration, Millipore) were coated with 5 μg ml −1 of anti-IgM (331, non-allotype-specific) or 1,000 HAU ml −1 purified A/Mem71. Plates were blocked with 4% bovine serum albumin (BSA) followed by addition of twofold serially diluted single-cell suspensions from various tissues in complete RPMI 1640 with 10% fetal bovine serum (FBS), which were incubated at 37 °C in a 5% CO 2 chamber for 16 h. Binding was revealed with biotinylated allotype-specific anti-IgM a (DS1.1) and anti-IgM b (AF6-78), followed by SA-HRP (Vector Labs). Spots were developed with 3-amino-9-ethylcarbazole (Sigma-Aldrich) and counted using an AID ELISpot Reader (Autimmun Diagnostika GmbH). Data are expressed as the number of IgM-secreting ASC per input cells. Magnetic enrichment of B-1 cells Pooled pleural or peritoneal lavage cells were harvested from 8 to 12 mice by flushing the cavity with 10 ml of PBS. Red blood cells were lysed by incubation with ACK lysis buffer and cells were stained as described for flow cytometry with combinations of the following antibodies (in-house generated or purchased as noted in flow cytometry description): CD90.2-biotin or CD4-, CD8a- and CD3-Biotin, with CD23-, F4/80-, CD49b- and Gr-1-Biotin and Streptavidin microbeads (Miltenyi Biotec), followed by negative depletion by autoMACS (Miltenyi Biotec). Purity of B-1 cells was >90%, as confirmed using flow cytometry with Streptavidin and CD19, IgM and IgD antibodies ( Supplementary Fig. 4a ). Quantitative RT–PCR RNA was isolated with the RNeasy micro-volume kit (Qiagen). Samples were stored in RNA Storage Buffer (Ambion) at −80 °C. cDNA was prepared by using random hexamers (Promega) with Super-Script II (Invitrogen). Amplification was performed with Clontech polymerase and commercial primer probes Mm00515153_m1 for Ifit1 , Mm00492606_m1 Ifit2 , Mm00487796_m1 Mx1 and Mm00484668_m1 for glyceraldehyde-3-phosphate dehydrogenase (GAPDH; Applied Biosystems), using the following amplification cycles on a Prism 7700 instrument (Applied Biosystems): 50 °C for 2 min, 95 °C for 10 min and 40 cycles of 95 °C for 15 s and 60 °C for 1 min. Data were normalized for expression relative to GAPDH. Indium-111 labelling MACS-enriched B-1 cells were labelled with 40 μCi of Indium-111 oxyquinolone for 10–15 min. After washing, cells were resuspended at 2 × 10 6 cells per 100 μl PBS and injected into the pleural cavity of anaesthetized recipient BALB/c mice. Mice were infected with A/Mem71 or mock-infected with PBS. Whole-body autoradiography was performed 3 days later. Scintillation fluid counting on various organs was performed to determine the level of radioactivity, and a standard curve of Indium-111-labelled B-1 cells was used to convert radioactivity to cell numbers. Intrapleural cell transfer AutoMACS-purified B-1 cells were stained with 0.25 μM caryboxyfluorescein succimidyl ester (CFSE; Invitrogen) or 1.25 μM eFluor 670 (eBioscience) cell-labelling dyes for 10 min at 37 °C, followed by triplicate washes in staining media containing 10% serum. Overall, 1 × 10 6 labelled cells were injected into the pleural cavity of anaesthetized C57BL/6-recipient mice in 100 μl sterile PBS, using a 28½G needle inserted through the right side of the diaphragm. At necropsy, tissues were processed to single-cell suspensions and fluorescently stained to identify B-1a cell populations using flow cytometry. Labelled B-1a cell populations were compared in tissues from A/Mem71-infected and control mice. B-1 cell shear flow adhesion assay B-1 cell adhesion properties were determined using a previously described microfluidic vascular-mimetic shear flow adhesion chamber [35] . Each chamber is composed of a mold containing four parallel channels placed over a coverslip. Shear flow is applied via connection to a syringe pump (Harvard Apparatus/Kent Scientific) and visualized using a × 20 phase contrast objective within an enclosed 37-°C incubator atop an inverted Nikon TE200 microscope. Overall, 5 × 10 6 purified B-1 cells ml −1 in buffer (0.5% BSA, 1 mM CaCl2 and 1 mM MgCl 2 in sterile PBS, pH 7.1) were infused through the channel at a rate of 0.75 dynes cm −2 (2.25 μl min −1 ) for 2 min. The rate was then increased to 3.3 dynes cm −2 (10 μl min −1 ) to disrupt weakly adhesive cells. Cellular arrest was measured on coverslips coated with the following ligands at previously titrated concentrations and blocked with Sea Block Blocking Buffer (Thermo Scientific) for 20 min before use: CXCL13 5 μg ml −1 (R&D Systems), ICAM-1 10 μg ml −1 (R&D Systems) and Fibrinogen 50 μg ml −1 (Abcam). For some experiments, B-1 cells were pre-treated with IFN-β (PBL Interferon Source) at 200 U ml −1 for 16 h and/or incubated with 10 μg ml −1 blocking antibodies (against CD11a (M17/4 BioLegend 101110), CD11b (M1/70 BioLegend 101214) and CD18 (M18/2 BioLegend 101409) at 37 °C for 20 min, while antibodies against CXCL13 100 μg ml −1 (R&D Systems AF470) were perfused through each chamber for 2–5 min to block the substrate. fMLP (Sigma-Aldrich) at 1 μM was added immediately before runs. Lovastatin (Calbiochem) at 100 μM was incubated with cells for 10 min. Eight-to-ten × 20 bright-field images were taken along the length of the flow chamber with an Orca-ER camera (Hamamatsu) coupled to a Nikon TE200 microscope running the SimplePCI 5.3 software (Compix) and processed for quantification using ImageJ (NIH). Intrapleural competition assay For studies comparing redistribution of two groups of cells within the same animal, B-1 cells were harvested from body cavities of CD11a−/−, CD11b−/−, Igha or C57BL/6 mice. Flow cytometry confirmed comparable frequencies of B-1 cells in cavities of integrin-deficient strains ( Supplementary Fig. 2d ). Comparisons between the groups of transferred cells were based on either Ig-allotype-specific identification or fluorescent labelling. For Ig-allotype-based assays, Ig-allotype differences in C57BL/6 (b-allo) or congenic Igha mice (a-allo) were used to distinguish between purified B-1 cells transferred into μMT mice lacking mature B cells. Cells were treated with combinations of IFN-β (PBL Interferon Source) 200 U ml −1 for 16 h in culture and some were treated in addition with 100 μM Lovastatin (Calbiochem) for 10 min before washing. For fluorescence-based assays, total cavity lavage or purified B-1 cells were stained with 0.25 μM CFSE (Invitrogen) or 1.25 μM eFluor 670 (eBioscience), both for 10 min at 37 °C followed by triplicate washes in staining media containing 10% serum and transfer into C57BL/6-recipient mice. For cell transfers, cells were mixed in equal proportions and 1 × 10 6 cells injected into the pleural cavity under general anaesthesia at various time points at or after A/Mem71 infection. At necropsy, tissues were processed to single-cell suspensions and fluorescently stained to identify B-1a cell populations using flow cytometry. The proportion of labelled B-1a cells was compared with the input proportion to generate a competitive index of recruitment efficiency compared with wild-type controls. For CD11b−/− studies, repeat experiments were performed using the opposite combinations of mouse strain and tracking dye and gave the same results. In vitro B-1 cell transwell migration assays Chemokine-mediated cell migration was evaluated using 5.0-μm pore Costar transwell plates (Corning Incorporated). Isolated pleural B-1 cells were plated overnight with mouse IFN-β. Cells were washed and 5 × 10 5 –1 × 10 6 cells plated in the upper portion of the transwell. Mouse CXCL13 chemokine (R&D Systems) at 1 μg ml −1 in RPMI/0.5% BSA was added to the lower portion of the transwell with or without anti-mouse CXCL13 (R&D Systems AF470) at 20 μg ml −1 . Each treatment group was plated in quadruplicate. After 3 h incubation at 37 °C, migrating cells in lower wells were removed and added to Polystyrene 15.0-μmicrosphere beads (PolySciences Inc.). Ratio of beads to cells was used to calculate cell numbers in the bottom chamber and normalize for cell loss during staining. Flow cytometry was used quantify % B-1 cell migration. Statistics Group sizes were based on preliminary studies and calculated to contain sufficient numbers of mice to reach statistical significance ( P ≤0.05) for group comparisons using power calculations. All data points were included in the study. Data were analysed with help of the Prism Software (GraphPad) using Student’s t- test, one sample t -test, one-or two-way analysis of variance to calculate statistical significance between groups. Statistical significance was assumed at * P ≤0.05, ** P ≤0.01, *** P ≤0.001, **** P ≤0.0001. How to cite this article: Waffarn, E. E. et al. Infection-induced type I interferons activate CD11b on B-1 cells for subsequent lymph node accumulation. Nat. Commun. 6:8991 doi: 10.1038/ncomms9991 (2015).